Ultrathin rhodium nanosheets Despite significant advances in the fabrication and applications of graphene-like materials, it remains a challenge to prepare single-layered metallic materials, which have great potential applications in physics, chemistry and material science. Here we report the fabrication of poly(vinylpyrrolidone)-supported single-layered rhodium nanosheets using a facile solvothermal method. Atomic force microscope shows that the thickness of a rhodium nanosheet is <4 Å. Electron diffraction and X-ray absorption spectroscopy measurements suggest that the rhodium nanosheets are composed of planar single-atom-layered sheets of rhodium. Density functional theory studies reveal that the single-layered Rh nanosheet involves a δ-bonding framework, which stabilizes the single-layered structure together with the poly(vinylpyrrolidone) ligands. The poly(vinylpyrrolidone)-supported single-layered rhodium nanosheet represents a class of metallic two-dimensional structures that might inspire further fundamental advances in physics, chemistry and material science. The discovery of ultrathin materials composed of single or few atomic layer(s), such as graphene [1] , molybdenum disulphide and boron nitride [2] , has aroused considerable recent interest. Such ultrathin materials exhibit fascinating properties such as high electron mobility, quantum Hall effects, extraordinary thermal conduction, magnetic resonant mode and superconductivity [3] , [4] , [5] , [6] , [7] , [8] . So far, the preparation of ultrathin materials with few atomic layers mainly relies on the material itself having a lamellar structure [9] , a feature that ensures the stability of their few- or even single-layer structures, because of the strong intra-layer chemical bonding and weak inter-layer interaction. In contrast, metal atoms have a strong preference for three-dimensional (3D) close-packed structures. Therefore, ultrathin metallic structures with a plethora of unsaturated atoms are difficult to stabilize and their synthesis remains challenging. More recently, the preparation of surfactant-capped Pd (ref. 10 ), Rh (ref. 11 ), and Ru nanoplates [12] with metal thicknesses of 1.8 nm, 1.3 nm and 1.5 nm, respectively, has been reported. In this work, we report the fabrication of poly(vinylpyrrolidone) (PVP)-supported single-layered rhodium nanosheets (Rh NSs) using a facile solvothermal method. We use aberration-corrected electronic microscopy, atomic force microscope (AFM) and X-ray absorption spectroscopy (XAS) to reveal that the Rh NSs are composed of planar single-atom-layer sheets of Rh. Density functional theory (DFT) investigations indicate that the single-layered Rh NS possesses a unique δ -bonding framework constructed from metallic – s hybrid orbitals, which stabilizes the single-layered structure together with the PVP ligands. The discovery of single-layered Rh NS points to the possibility of fabricating similar structures for other metals. Further investigations of such materials might lead to vital advances in physics, chemistry and material science. Synthesis and characterizations Herein, using a solvothermal synthetic approach we obtained semi-transparent Rh NSs with an edge length of ca . 500–600 nm in the presence of PVP in high yield (see Fig. 1a,b , and Methods for details). These nanosheets are highly sensitive to electron beam irradiation in high-resolution transmission electron microscopy (HRTEM) (see Supplementary Fig. 1 ), suggesting an ultrathin Rh structure. Moreover, X-ray diffraction pattern of the sample showed no diffraction peaks (see Supplementary Fig. 2 ), also indicative of an ultrathin nature. Energy-dispersive X-ray studies (see Supplementary Fig. 3 ) indicate that the individual NSs are composed of Rh NSs capped with PVP, which is further verified by Fourier transform infrared spectroscopy (FTIR, Supplementary Fig. 4 ). 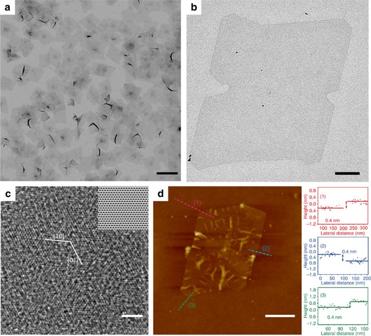Figure 1: Characterization of ultrathin Rh NSs. (a) Low-magnification TEM image of the PVP-capped Rh NSs. Scale bar, 1 μm. (b) High-magnification TEM image of the PVP-capped Rh NSs. Scale bar, 100 nm. (c) Aberration-corrected microscopy image of a PVP-capped Rh NS (inset, the corresponding filtered image using the crystallographic average method to improve signal-to-noise ratio). Scale bar, 2 nm. (d) AFM image and the corresponding height profiles of a bare Rh NS. Scale bar, 200 nm. Figure 1: Characterization of ultrathin Rh NSs. ( a ) Low-magnification TEM image of the PVP-capped Rh NSs. Scale bar, 1 μm. ( b ) High-magnification TEM image of the PVP-capped Rh NSs. Scale bar, 100 nm. ( c ) Aberration-corrected microscopy image of a PVP-capped Rh NS (inset, the corresponding filtered image using the crystallographic average method to improve signal-to-noise ratio). Scale bar, 2 nm. ( d ) AFM image and the corresponding height profiles of a bare Rh NS. Scale bar, 200 nm. Full size image Structural determination In order to minimize irradiation damage to the PVP-capped Rh NSs during electron microscopy characterization, low electron exposures were employed with concomitant lower signal-to-noise ratio than that observed under standard imaging conditions. Aberration-corrected electron microscopy with optimum focus was used to improve the signal-to-noise ratio (see Methods for details). The object plane of the objective lens was set to the mid-plane of the carbon support to reduce the noise from the support [13] . Accordingly, the carbon support was in the Gauss focus and its contrast was minimized, whereas the PVP-capped Rh NSs were close to the Scherzer focus, giving a high contrast. Experimental images (see Fig. 1c ) were processed using the crystallographic average method to further improve the signal-to-noise ratio (see Fig. 1c , inset). The images reveal the single-crystalline nature of Rh NS, which possesses a hexagonal structure, with a lattice parameter of ca . 2.6 Å, close to the atomic distance of Rh (2.69 Å) in the (111) plane of the bulk Rh phase. From the viewpoint of symmetry, both face-centered-cubic (fcc) and hexagonal-close-packed (hcp) structures could give a hexagonal lattice—in the [111] and [0001] directions, respectively. In the [111] zone axis of fcc Rh, however, the projected structure would show a lattice parameter of 1.55 Å, which is not the case here. To evaluate the thickness of Rh NS, the PVP capping on the surface of Rh NSs was removed by calcinating the PVP-capped Rh NSs supported on silica wafer in flowing O 2 at 600 °C, which led to the formation of silica wafer-supported Rh NS (see Methods for details). AFM imaging of the Rh NS supported on silica wafer shows that the sheet-like features were well preserved compared with TEM images (see Fig. 1a,b ) upon above treatment. Section analysis and height profile (see Fig. 1d ) reveal that the height of Rh NS is ca . 4 Å. Given the Rh atomic radius of 1.73 Å, this Rh NS likely consists of only single Rh atomic layer in thickness, which is also confirmed by HRTEM (see Supplementary Fig. 5 and Methods for details). Analysis of the intensity profiles of electron diffraction patterns has been demonstrated to be a valid and important method for the accurate determination of the thickness of a graphene sheet [14] . For instance, in single-layered graphene the intensities of diffraction spots in the outer hexagons are comparable to those in the inner hexagons, whereas for multilayers the diffraction spots in the outer hexagons are more intense [15] . In the case of PVP-capped Rh NS, since the thickness of bare Rh NS is less than the extinction distance in electron dynamical diffraction—which is typically tens of nanometres—kinematical electron diffraction was performed. 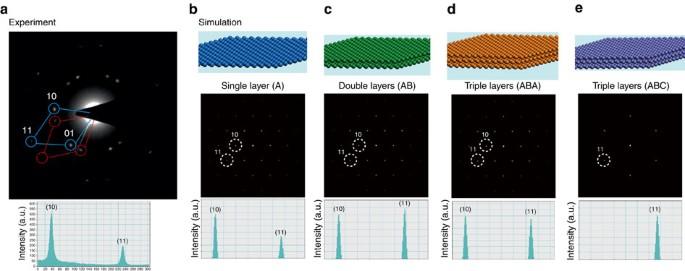Figure 2: Experimental and simulated electron diffraction patterns. (a) Experimental electron diffraction pattern and the corresponding intensity profiles of the PVP-capped Rh NSs. Simulated electron diffraction patterns and the corresponding intensity profiles of (b) single layer, (c) double layers, (d) triple layers in a hcp ABA stacking sequence and (e) triple layers in an fcc ABC stacking sequence of Rh crystals. The intensity profiles of the diffraction patterns show the relative intensities of the (10) and (11) diffraction beams. The letters ‘A’, ‘B’ and ‘C’ denote the relative positions of the atomic layers within the sheet plane. Figure 2a shows a typical experimental electron diffraction pattern and the corresponding intensity profile of the PVP-capped Rh NSs. Two sets of diffraction spots obtained from two PVP-capped Rh NSs (rotated by 16 degree with respect to each other) are labelled by the full (blue) cycles and dotted (red) cycles in Fig. 2a . Diffracted intensity profiles taken along the full (blue) line denoted by (10) and (11) directions showed clearly that the intensity of the spot in the inner hexagon is twice the intensity of the spot in the outer hexagon. The same goes for the other set of diffraction spots labelled by dotted (red) cycles. For a quantitative comparison between the experimental and simulated diffraction patterns, JEMS software was used to obtain simulated diffraction patterns for candidate structures with thicknesses up to six Rh atomic layers (see Fig. 2b–e and Supplementary Fig. 6 ). The corresponding intensity profiles for the simulated diffraction patterns are also given for comparison. It is noteworthy that the intensity of the inner spot (10) is twice the intensity of the outer spot (11) only for the simulated diffraction patterns for single-layered Rh (see Fig. 2b ), which is consistent with the experimental diffraction patterns (see Fig. 2a ). For the other multi-layered structures, the calculated intensities do not match the experimental pattern: for the double layered structures (AB) or hcp-type triple layers (ABA) the beams (10), (01) and (11) have similar intensities, and in the fcc-type triple layers (ABC) the (10) and (01) beams are absent, corresponding to an image of a hexagonal lattice with a lattice constant of 1.55 Å. Since the calculated patterns for lattices with more than three layers do not match the experimental pattern either, a planar single-atom layer sheet of Rh capped with PVP is indicated for the nanosheet. Figure 2: Experimental and simulated electron diffraction patterns. ( a ) Experimental electron diffraction pattern and the corresponding intensity profiles of the PVP-capped Rh NSs. Simulated electron diffraction patterns and the corresponding intensity profiles of ( b ) single layer, ( c ) double layers, ( d ) triple layers in a hcp ABA stacking sequence and ( e ) triple layers in an fcc ABC stacking sequence of Rh crystals. The intensity profiles of the diffraction patterns show the relative intensities of the (10) and (11) diffraction beams. The letters ‘A’, ‘B’ and ‘C’ denote the relative positions of the atomic layers within the sheet plane. Full size image Although HRTEM, AFM and electron diffraction analysis all provide evidence of an ultrathin or even single-atom layer structure of Rh NS, the conclusion is only valid for the limited number of Rh NSs studied in the microscope. Inasmuch as XAS is a powerful technique for studying the atomic structure of nanomaterials [16] due to its ability in providing a statistical result for a bulk sample, it was used to elucidate the local coordination environment of Rh atoms and to determine the thickness of Rh NS on a macroscopic level (see Methods for details). For comparison the XAS spectra of Rh foil and PVP-capped 3D Rh nanoparticles (Rh NPs, with an average size of ~13.5 nm, see Supplementary Fig. 7 for the TEM image and Methods for synthesis) were also measured. The X-ray absorption fine structure (XAFS) spectra and k-space spectra (see Fig. 3a,b , respectively) of the PVP-capped Rh NPs and PVP-capped Rh NSs are similar and closely resemble that of Rh foil, but with reduced oscillations in the case of the PVP-capped Rh NSs. Indeed, in the Fourier-transformed extended XAFS (EXAFS) spectra (see Fig. 3c ), the intensity of the peak at 2.37 Å, assigned to the first shell Rh–Rh scattering, decreases in the order Rh foil>PVP-capped Rh NP ≫ PVP-capped Rh NS. This result indicates that the Rh atoms in the PVP-capped Rh NSs possess a coordination environment that is different from that of the Rh atoms in the PVP-capped Rh NPs and foil samples. The Rh–Rh coordination number (CN) is sensitive to both particle size and morphology at the nanoscale. The coordination environments in structures with different number of Rh layers are illustrated schematically in Fig. 3d . For a single-layered, close-packed, infinite Rh structure, the first shell CN is 6, as each Rh atom is surrounded by 6 other Rh atoms. Double- and triple-layered Rh structures have higher CNs (9 and 10 respectively) due to the additional inter-layer Rh–Rh coordination. For close-packed NPs, the CN is also high—at least 9 for NPs with a particle size >2 nm (ref. 17 ). From curve fitting ( Table 1 ), the PVP-capped Rh NPs have a CN of 10.4±0.8, in agreement with the expected value. In contrast, a CN of only 6.4±0.7 is obtained for the PVP-capped Rh NSs, fitting well with the CN of a single-layered system. In addition, the average Rh–Rh bond length in PVP-capped Rh NSs, estimated as 2.692±0.004 Å from the XAS spectra, is similar to that of Rh foil (2.687±0.003 Å), indicating the Rh NS is composed of close-packed Rh atoms. 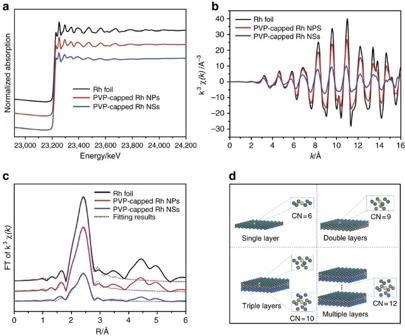Figure 3: Structure determination of ultrathin Rh NSs by XAS. (a) Normalized Rh K-edge EXAFS spectra of Rh foil, PVP-capped Rh NPs, and PVP-capped Rh NSs. (b) k3-weighted Rh K-edge k-space oscillations of Rh foil, PVP-capped Rh NPs and PVP-capped Rh NSs. (c) Fourier-transformed spectra of k3-weighted Rh K-edge EXAFS of Rh foil (solid black line), PVP-capped Rh NPs (solid red line) and PVP-capped Rh NSs (solid blue line) and corresponding curve-fitting results (dotted purple lines). (d) Schematic illustration of the coordination states with CN of Rh NS with single, double, triple and multiple layers with an exposed Rh (111) lattice plane (the yellow balls indicate the ‘core’ Rh atoms). Figure 3: Structure determination of ultrathin Rh NSs by XAS. ( a ) Normalized Rh K-edge EXAFS spectra of Rh foil, PVP-capped Rh NPs, and PVP-capped Rh NSs. ( b ) k 3 -weighted Rh K-edge k-space oscillations of Rh foil, PVP-capped Rh NPs and PVP-capped Rh NSs. ( c ) Fourier-transformed spectra of k 3 -weighted Rh K-edge EXAFS of Rh foil (solid black line), PVP-capped Rh NPs (solid red line) and PVP-capped Rh NSs (solid blue line) and corresponding curve-fitting results (dotted purple lines). ( d ) Schematic illustration of the coordination states with CN of Rh NS with single, double, triple and multiple layers with an exposed Rh (111) lattice plane (the yellow balls indicate the ‘core’ Rh atoms). Full size image Table 1 Structural parameters obtained from the curve-fitting analysis of the EXAFS spectra shown in Fig. 3. Full size table In addition, we analysed the EXAFS data by taking into account the Rh–O contribution. Listed in Supplementary Fig. 8 and Supplementary Table 1 are the Fourier-transformed EXAFS spectra of Rh NS in the range of 2–13 inverse Angstroms, and the fitting results with and without considering a Rh–O shell. We also present in Supplementary Fig. 9 and Supplementary Table 2 the Fourier-transformed EXAFS spectra of Rh foil and Rh NS in the range of 2–8 inverse Angstroms and their corresponding fitting results. Clearly incorporating a Rh–O shell significantly improved the fitting quality, when the k-range is reduced to 2–8 inverse Angstroms, suggesting that the Rh–O bonds plausibly exist on Rh nanosheets. In this case, the CN of Rh–Rh is 5.6 ±1.0, essentially the same as the single Rh–Rh shell fitting results presented in our work. The CN of Rh–O is 1.0 ±0.6. Here the large uncertainty is simply because the number of independent fitting parameters exceeds the statistic limitation. Electronic structures and stability In order to elucidate the nature of the unexpected stability of the prepared single-layered Rh NSs, DFT studies (see Methods for details) were carried out on finite planar Rh x ( x =7, 19, 37, 61) clusters with D 6h point-group symmetry (see Supplementary Fig. 10 ) and an infinite single-layered slab. 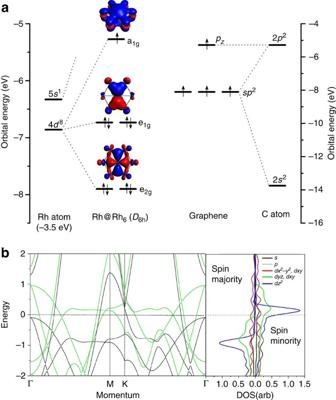Figure 4: DFT calculations of single-layered structure of Rh atoms. (a) Rh 4d orbitals split into e2g(dxy,d–), e1g(dxz,dyz) and a1g() species upon interacting with six peripheral Rh atoms in a Rh7(D6h) cluster (left). The highest a1gorbital forms the delocalized δ-bonding mentioned in the text. The Kohn–Sham orbitals are plotted with isosurface value=0.03 atomic units. The energy levels of the central Rh atom in a vacuum are shifted by −3.5 eV for clarity. C (2s22p2) forms threesp2hybrid orbitals and onepzorbital during the formation of graphene (right). (b) The band structures (left) and the local spin-orbital density of states (LDOS) (right) of a single-layered Rh NS-derived from a periodic slab model. The black and green lines in the band structures correspond to the spin-majority and spin-minority bands, respectively. Theσ-,π- andδ-contributions are shown in red, green and blue colours in the LDOS, respectively. Figure 4a compares the bonding pattern of C atom in graphene and Rh atom in Rh NSs. The calculated band structures and local density of states for the single-layered slab model are shown in Fig. 4b . Our calculated spin densities on the central atoms of the clusters and the magnetic moment in the periodic slab are close to 1 for each Rh atom. The calculated nucleus-independent chemical shift value at 1 Å above the centre of the Rh 7 hexagon is −12.04 p.p.m., which is close to that for benzene (−11.2 p.p.m.) and other polybenzenoid hydrocarbons of graphene fragments [18] . Figure 4: DFT calculations of single-layered structure of Rh atoms. ( a ) Rh 4d orbitals split into e 2g ( d xy , d – ), e 1g ( d xz , d yz ) and a 1g () species upon interacting with six peripheral Rh atoms in a Rh 7 (D 6h ) cluster (left). The highest a 1g orbital forms the delocalized δ-bonding mentioned in the text. The Kohn–Sham orbitals are plotted with isosurface value=0.03 atomic units. The energy levels of the central Rh atom in a vacuum are shifted by −3.5 eV for clarity. C ( 2s 2 2p 2 ) forms three sp 2 hybrid orbitals and one p z orbital during the formation of graphene (right). ( b ) The band structures (left) and the local spin-orbital density of states (LDOS) (right) of a single-layered Rh NS-derived from a periodic slab model. The black and green lines in the band structures correspond to the spin-majority and spin-minority bands, respectively. The σ -, π - and δ -contributions are shown in red, green and blue colours in the LDOS, respectively. Full size image Catalytic properties Hydrogenation [19] and hydroformylation [20] reactions represent important industrial processes, producing key feedstocks for the synthesis of fine chemicals. The commonly used catalyst for these reactions is Rh metal [21] , [22] . However, given its limited reserves and high price compared with other noble metals, it is important to design Rh catalysts with high atomic efficiency. One way of doing this is to fabricate single-layer materials with 100% exposed Rh atoms with unsaturated coordination. To investigate the catalytic properties of PVP-capped Rh NSs, hydrogenation of phenol and hydroformylation of 1-octene were employed as probe reactions. Rh NPs and commercial Rh/C (see Supplementary Figs 6 and 11 , respectively) were chosen as the benchmark catalysts (see Methods for details). 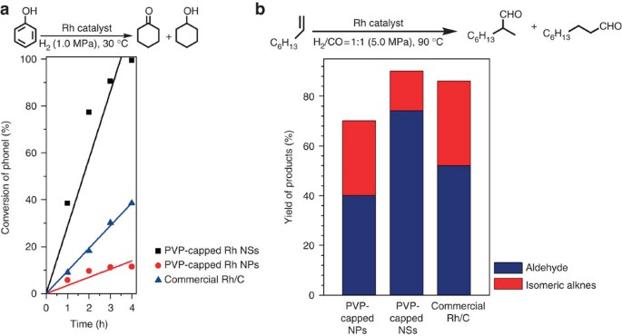Figure 5: Comparison of catalytic ability of PVP-capped Rh NSs, PVP-capped Rh NPs, and commercial Rh/C. (a) Hydrogenation of phenol and (b) hydroformylation of 1-octene. Reaction conditions and other details are shown inSupplementary Tables 3 and 4. Figure 5a displays a comparison of the conversion of phenol over reaction time catalysed by different Rh catalysts. The best performance was achieved with PVP-capped Rh NSs, which gave >99.9% conversion within 4 h at near room temperature (30 °C) under low H 2 pressure (1.0 MPa) and showed an activity that was, respectively, four- and seven times greater than those of commercial Rh/C and PVP-capped Rh NPs (based on the conversion at 1 h). Without further optimization, all the catalysts show comparable selectivity to cyclohexanone and cyclohexanol (see Supplementary Table 3 ). Especially, in the hydroformylation of 1-octene, when compared with commercial Rh/C and PVP-capped Rh NPs, our PVP-capped Rh NSs was found to give both superior catalytic activity and selectivity towards the target product (aldehyde) under mild reaction conditions (see Fig. 5b and Supplementary Table 4 ). Since surface atoms are important in heterogeneous catalysis [23] , a high proportion of surface atoms will enhance the efficiency of catalytic reactions. The proportion of surface Rh atom in the PVP-capped Rh NSs is 100%, whereas this is not possible in the commercial Rh/C or PVP-capped Rh NPs (see Supplementary Figs 12 and 13 , Supplementary Table 5 and Supplementary Note 1 for more details). As a result, a full exposure of Rh atoms in the PVP-capped Rh NSs accounts for the largely enhanced catalytic activity. Figure 5: Comparison of catalytic ability of PVP-capped Rh NSs, PVP-capped Rh NPs, and commercial Rh/C. ( a ) Hydrogenation of phenol and ( b ) hydroformylation of 1-octene. Reaction conditions and other details are shown in Supplementary Tables 3 and 4 . Full size image We have successfully synthesized single-layered Rh NSs capped with PVP. HRTEM, AFM, electron diffraction analysis and XAS studies suggest that the Rh NSs contain single-atom layer of Rh. It is not unreasonable to expect that our synthetic approach might be extended to the preparation of surfactant-capped single-atom-layered sheets of other metals. These single-layered NSs of metals might find potential applications in catalysis and material physics. Metals with an fcc or hcp structure have non-directional 3D metallic bonding, rather different from layer-structured materials such as graphene with strong in-plane σ -bonding together with π -bonding by the perpendicular orbitals [2] . As shown in Fig. 4a , in graphene each C atom has half-filled ( sp 2 ) [3] hybrid orbitals that form the σ -skeleton and a ( p z ) [1] orbital that form the familiar delocalized π -bonding framework. Our calculation show that in the single-layered Rh sheet each Rh atom has fully filled ( d xy , d – ) [4] and ( d xz , d yz ) [4] orbitals available for weak σ - and π -type interactions with surrounding Rh atoms, and a half-filled () [1] for shoulder-to-shoulder δ -type interactions with other Rh centres [24] . These results agree with our calculated spin densities on the central atoms of the clusters and the magnetic moment in the periodic slab. As a result of the significant –s orbital mixing, a conjugated δ -bonding framework composed of the –s hybrid orbitals of the Rh atoms is generated, which is responsible for electron delocalization throughout the whole cluster (see Fig. 4a ). The calculated band structures and local density of states (see Fig. 4b ) for the single-layered slab model also show that in the single-layered Rh sheet the bonding and antibonding σ - and π -interactions nearly cancel out, while the 4 (and 5s ) orbitals from all the Rh centres form spin-polarized bands with a net bonding effect, which contribute to the high surface energy and electron delocalization. Clearly the δ -bonding delocalized in the single-layered Rh sheet contributes to its stability. The calculated nucleus-independent chemical shift value indicates that the single-layered Rh sheet has quasi-aromatic stability and a diatropic ring current in a magnetic field. On the other hand, the formation of conjugated δ -bonding partially saturates the dangling bonds, thereby to a certain extent decreasing the surface energy of the single-layered Rh. Despite the conjugated δ -bonding contribution to the stability of the Rh sheet, a bare Rh sheet is likely less stable than a 3D packed structure, thus requiring further stabilization through surface ligands such as PVP [25] . Indeed, while the calculated phonon spectrum of the single-layered Rh NSs show non-negligible imaginary frequencies for the out-of-plane motions of Rh atoms (see Supplementary Fig. 14a ), these imaginary frequency modes are largely suppressed upon adsorption of simplified PVP ligands (2-pyrrolidone molecule), with the imaginary frequencies significantly reduced to within those of the numerical noise (see Supplementary Fig. 14b ). Moreover, the surface energy decreases from 0.126 for bare Rh sheet to 0.071 eV Å −2 for the simplified PVP-covered ones. These results are in line with the experimental observation that the single-layered Rh NSs are formed with the help of PVP capping. Consistent with these theoretical results, our experiment shows that fabrication in the absence of PVP yields aggregates of Rh NSs (see Supplementary Fig. 15 ). Because of the unique bonding of the Rh atoms, the resulting nanoscale materials may find applications in electronics, magnetic devices and catalysis. Based on the analogy with graphene, we propose to call the single-layered metal nanosheet as ‘metallene’. Reagents Rh(III) acetylacetonate (Rh(acac) 3 , 99%), commercial Rh black, commercial Rh/C (5% metal) were purchased from Alfa Aesar. Poly(vinylpyrrolidone) (PVP, MW=30,000), L -ascorbic acid (AA), benzyl alcohol, formaldehyde, phenol, cyclohexanone, cyclohexanol and 1-octene were purchased from Sinopharm Chemical Reagent Co. Ltd. (Shanghai, China). All regents were used as received without further purification. Synthesis of PVP-capped ultrathin Rh nanosheets Rh(acac) 3 (8.0 mg), PVP (MW=30,000, 120.0 mg) were dissolved in benzyl alcohol (3 ml) and formaldehyde (3 ml). The mixture was stirred vigorously for 1 h and then transferred to a Teflon-lined stainless steel autoclave. The autoclave was sealed and maintained at 180 °C for 8 h and then cooled to room temperature. The resulting black product was precipitated with acetone (10 ml), separated in a centrifuge and washed three times with ethanol (10 ml) and finally dried under vacuum. Synthesis of PVP-capped Rh nanoparticles Rh(acac) 3 (8.0 mg), PVP (MW=30,000, 120.0 mg) and AA (40 mg) were dissolved in benzyl alcohol (6 ml). The mixture was stirred vigorously for ~1 h and then transferred to a Teflon-lined stainless steel autoclave. The autoclave was sealed and maintained at 180 °C for 8 h and then cooled to room temperature. The resulting black product was precipitated with acetone (10 ml), separated in a centrifuge and washed three times with ethanol (10 ml) and finally dried under vacuum. Transmission electron microscope analysis Transmission electron microscope (TEM) and HRTEM studies were performed on a Hitachi model H-800 TEM or JEOL-2010F HRTEM operating at 200 kV. HRTEM analysis HRTEM images were recorded on a JEOL JEM-2100 microscope using bright-field microscopy at an accelerating voltage of 200 kV. Aberration-corrected electronic microscopy analysis Aberration-corrected electronic microscopy observations were performed on an FEI Titan 80-300 TEM equipped with a spherical aberration (Cs) corrector as the objective lens. The information limit of the microscope is 0.08 nm. The images were taken using the negative-Cs imaging technique, which was shown to give high contrast and low noise. The images were taken at a high tension of 300 kV, with the spherical aberration set at around –13 μm. Because of the high sensitivity of the PVP-capped Rh NSs to irradiation by the electron beam, the electron exposure was kept as low as possible during the experiments. Kinematical electron diffraction patterns were simulated using MacTempas and JEMS softwares. For the PVP-capped Rh NSs, dynamic diffraction was neglected. AFM analysis AFM analysis was performed in tapping mode in air with a Multimode Nanoscope IIIa SPA (Veeco Instruments, Bruker). Ultrasharp cantilevers with a diamond-like carbon tip (NSG01, NT-MDT, Russia) were used. The image was flattened using the NanoScope Analysis software (version 1.40). A silicon wafer with thermal oxide layer of 2.850 Å in thickness (Silicon Valley Microelectronics, Inc. USA) was used. The surfactant PVP could be removed after high temperature oxygen pretreatment reactions, as reported by Somorjai et al. [26] , [27] , [28] In our study, The AFM sample was prepared by the following procedures: PVP-capped Rh NSs was initially dispersed in ethanol and then placed dropwise on the silicon wafer. The formed silica wafer supported sample was dried in air and subsequently calcinated in tubular furnace in flowing O 2 from room temperature to 600 °C with a heating rate of 0.5 °C min −1 , after which the temperature was maintained at 600 °C for 1 h. After this silica wafer-supported sample was cooled down to room temperature, it was treated in flowing H 2 at 600 °C for 2 h. After these procedures, the PVP surfactant was removed by the oxidation of O 2 , leaving Rh NSs supported on silica wafer, which was then used for the AFM analysis. Observation of cross-section of Rh nanosheets The PVP-capped Rh NSs were dispersed in 1 ml of epoxy resin embedding medium (Epon 812). After 15-min ultrasonic re-dispersion, a drop of 2,4,6-Tris(dimethylaminomethyl)phenol (DMP-30) was added as a hardener. Subsequently, the mixture was dried at 80 °C in an oven for 24 h. Ultrathin sections (~30 nm thickness) were prepared using a Diatome diamond knife on a Leica EM UC6 ultramicrotome, and transferred onto Cu grids with a lacey carbon supporting film. The embedding medium stabilized the Rh NSs against electron irradiation and simultaneously fixed the Rh NSs in the hard mixture in random directions. By using this method, the morphology of ultrathin Rh NSs was maintained under electron irradiation to some extent and the cross-section images could be observed. Supplementary Fig. 5 shows the cross-section of an assembly of Rh NSs embedded in an epoxy resin, in which three Rh NSs (shown by arrows) were found to pack parallel to each other with a distance of ca . 7.6 Å, forming a lamellar structure. Each sheet has a thickness of ~3.6 Å, an order of magnitude smaller than the thickness of most reported ultrathin metallic nanosheets. XAS analysis XAS experiments were performed at Photon Factory, KEK, Tsukuba, Japan, under the approval of the Photon Factory Advisory Committee (proposal no. 2012G601). The X-ray energy was calibrated using an inflection point of Rh foil in the X-ray absorption near edge structure. The XAS measurements of the Rh K-edge of PVP-capped Rh NSs and PVP-capped Rh NPs dispersed in ethanol (Rh= ca . 10 mg ml −1 ) were carried out at room temperature in transmission mode, by employing a Si(311) crystal for the monochromatic synchrotron radiation. Data reduction of the XAFS spectra was conducted with Athena and Artemis included in the Ifeffit package. The k 3 -weighted EXAFS oscillation in the range 2–13 Å −1 was Fourier-transformed and curve-fitting analysis was performed in the range 1.8–2.8 Å in R space. For curve-fitting analysis, the backscattering factor and the phase shift of the scattering path were calculated with FEFF6L using the crystal structure of Rh metal. The amplitude reduction factor was also estimated by fitting the spectrum of Rh foil with the parameters calculated with FEFF. Details of theoretical calculations Cluster models: DFT calculations were carried out on a series of planar Rh x ( x =7, 19, 37, 61) clusters with D 6h point-group symmetry (see Supplementary Fig. 10 ) by using the Amsterdam Density Functional code (ADF 2010.02). [29] , [30] , [31] The PBE functional [32] and a Slater-type-orbital (STO) basis sets with quality of double-ζ (DZ) and triple-ζ plus polarization functions (TZP) [33] were used for all atoms. The frozen core approximation was employed for inner shells [ 1s 2 – 3d 10 ] of Rh. Numerous calculations were performed to determine the spin multiplicities of these clusters. The smallest Rh 7 cluster was found to have 13 unpaired electrons, with roughly two spins on the peripheral Rh atoms and one spin on the central Rh atom. Figure 4a shows the orbital splittings of C in graphene as sp 2 + p z and Rh in the Rh 7 sheet as σ ( d xy , d – ), π ( d xz , d yz ) and δ () species, which are mainly composed of 4d orbitals of the central Rh atom. The central Rh atom of the Rh 7 cluster tends to have similar properties to those of an arbitrary atom of a single-layered Rh (111) surface. Owing to the ligand field in the D 6h point group, the d orbitals of the central Rh atom split into three groups with irreducible representations e 2g , e 1g and a 1g , mainly participating in the corresponding molecular orbitals displayed in Fig. 4a . Note that the highest a 1g -type orbitals from each Rh atom form the delocalized δ -bonding mentioned in the text, which involves the –s hybrid orbital of Rh atoms. Slab model for single-layered Rh The periodic DFT calculations were performed using the Vienna ab initio simulation package (VASP) [34] . The spin-polarized generalized gradient approximation with the PBE functional [32] and the projector augmented wave (PAW) method [35] with a cutoff energy of 400 eV were used. A p (3 × 3) supercell was adopted for single-layered Rh with the vacuum spacing set at least 28 Å. Integration over the Brillouin zone was achieved using the Monkhorst–Pack scheme with 11 × 11 × 1 and 33 × 33 × 1 meshes for structural optimizations and electronic structure calculations, respectively. The phonon spectra were calculated on a Rh nanosheet capped with simplified PVP ligands (2-pyrrolidone molecules) within the usual harmonic approximation. Procedure for hydrogenation of phenol In a typical catalytic reaction, phenol (0.1 mmol), ZnCl 2 (0.01 mmol), 0.64 mol % Rh catalysts (PVP-capped Rh NSs, PVP-capped Rh NPs or commercial Rh/C) suspension in CH 2 Cl 2 (1 ml) were placed in an autoclave. To remove the air from the reaction system, the autoclave was purged three times with H 2 . Subsequently, the autoclave was pressurized with H 2 (1.0 MPa) and the reaction mixture was stirred at 600 r.p.m. at 30 °C for the required time. Procedure for the hydroformylation of 1-octene In a typical catalytic reaction, 1-octene (5.0 mmol) and 0.02 mol % Rh catalysts (PVP-capped Rh NSs, PVP-capped Rh NPs or commercial Rh/C) suspension in isopropanol (15 ml) were placed in an autoclave. To remove the air from the reaction system, the autoclave was purged three times with N 2 and then three times with H 2 /CO (1:1) mixed gas. Subsequently, the autoclave was pressurized with H 2 /CO (1:1, 5.0 MPa) mixed gas and the reaction mixture was stirred at 580 r.p.m. at 90 °C for 3 h. How to cite this article: Duan, H. et al. Ultrathin rhodium nanosheets . Nat. Commun. 5:3093 doi: 10.1038/ncomms4093 (2014).